Cancer cells that survive radiation therapy acquire HIF-1 activity and translocate towards tumour blood vessels Tumour recurrence frequently occurs after radiotherapy, but the characteristics, intratumoural localization and post-irradiation behaviour of radioresistant cancer cells remain largely unknown. Here we develop a sophisticated strategy to track the post-irradiation fate of the cells, which exist in perinecrotic regions at the time of radiation. Although the perinecrotic tumour cells are originally hypoxia-inducible factor 1 (HIF-1)-negative, they acquire HIF-1 activity after surviving radiation, which triggers their translocation towards tumour blood vessels. HIF-1 inhibitors suppress the translocation and decrease the incidence of post-irradiation tumour recurrence. For the first time, our data unveil the HIF-1-dependent cellular dynamics during post-irradiation tumour recurrence and provide a rational basis for targeting HIF-1 after radiation therapy. Aberrantly accelerated proliferation and metabolism are typical characteristics of cancer cells [1] , which lead to an imbalance between oxygen supply and oxygen consumption in a solid tumour and cause a tumour-specific microenvironment, hypoxia [2] , [3] . Clinical studies using a computerized polarographic needle electrode have revealed that in malignant tumours, such as uterine cervix cancer, head-and-neck cancer and breast cancer, overall median partial oxygen pressure (pO 2 ) is about 10 mm Hg and the overall hypoxic fraction (pO 2 <or=2.5 mm Hg) is ~25% (ref. 4 ). In contrast, pO 2 values lower than 12.5 mm Hg were not found in normal tissues, such as normal breast tissue [5] . Immunohistochemical analyses with markers have clarified the intratumoural localization of hypoxia in detail [6] . Because of the limited distance molecular oxygen can diffuse, most malignant tumours grow individually as a conglomerate of so-called 'micro tumour cords', in each of which a blood vessel is surrounded by well-oxygenated (normoxic), then oxygen-insufficient (hypoxic), and finally oxygen-depleted (anoxic/necrotic) cancer cells [2] , [7] . In addition to such chronic hypoxia, acute hypoxia is known to develop even proximal to blood vessels as a result of the transient functional failure/occlusion of blood vessels [8] , [9] . Hypoxia achieves many of its effects through the activation of a transcription factor, hypoxia-inducible factor 1 (HIF-1). HIF-1 is a heterodimer composed of an α-subunit (HIF-1α) and a β-subunit (HIF-1β), and its activity is mainly dependent on the stability and modification of HIF-1α [10] . Under normoxic conditions, the oxygen-dependent degradation (ODD) domain of HIF-1α is hydroxylated by prolyl hydroxylases and ubiquitinated by a pVHL-containing E3 ubiquitin ligase, resulting in rapid proteolysis of the subunit [11] , [12] . Under hypoxic conditions, however, HIF-1α is stabilized and interacts with HIF-1β [10] . The resultant heterodimer, HIF-1, binds to its cognate enhancer sequence, the hypoxia-responsive element (HRE), and induces the expression of various genes responsible for 'adaptation of cellular metabolism to hypoxia (the switch from oxidative to anoxic respiration) (ref. 13 )', 'escape from hypoxia (invasion and metastasis of cancer cells) (refs 14 , 15 )', and 'improvement of hypoxia (angiogenesis) (refs 16 , 17 )'. The radioresistance of individual cancer cells is known to be influenced by various intrinsic and extrinsic factors, and therefore is highly dissimilar in diverse and heterogeneous tumour microenvironments. Accumulated evidence has suggested that one of the most influential factors is hypoxia [2] , [3] , [18] , [19] . Depletion of oxygen is reported to directly disturb radiation-induced production of reactive and cytotoxic species (chemical oxygen effect) [8] , [19] . Moreover, hypoxia is known to induce tumour radioresistance through the activation of HIF-1 (biological oxygen effect) [20] , [21] , [22] , [23] . Consistent with these findings, there is clinical evidence that both the size of the intratumoural hypoxic fraction and the level of HIF-1α correlate with a poor prognosis after radiation therapy [4] , [24] , [25] . However, regarding the dynamic changes of the tumour microenvironment during tumour growth and after radiation therapy, problems in hypoxia-mediated radioresistance seem to be more complicated. Immunohistochemical analysis with both an anti-HIF-1α antibody and a hypoxia marker, pimonidazole, recently revealed that HIF-1α-positive cells are not necessarily stained with pimonidazole [26] , [27] . Namely, in some types of malignant tumours, chronic hypoxia can be histologically categorized into two sectors: HIF-1α-positive/pimonidazole-negative and pimonidazole-positive/HIF-1α-negative. This fact has repeatedly been confirmed in various human tumours as well as tumour xenografts [26] , [27] , [28] . Moreover, immunostaining combined with optical real-time imaging for HIF-1 activity revealed that ionizing radiation dramatically alters the distribution of oxygen and nutrients in a solid tumour, triggering a transient decrease and subsequent increase in intratumoural HIF-1 activity [20] , [29] , [30] , [31] . Because of these spatiotemporal complexities, how, when, and where the radiochemical and radiobiological mechanisms function in tumour radioresistance are largely unknown. Moreover, the characteristics, intratumoural localization, and post-irradiation dynamics of radioresistant cancer cells have not been clarified yet. To address these issues, we established a strategy to separately tag HIF-1α-positive/pimonidazole-negative cells and pimonidazole-positive/HIF-1α-negative cells at a precise window in time. Subsequent cell-tracking experiments revealed that the pimonidazole-positive/HIF-1α-negative cancer cells survive radiation better than their counterparts. Moreover, we demonstrate for the first time, that the surviving cells acquire high levels of HIF-1 activity in areas of radiation-induced reoxygenation and translocate towards tumour blood vessels after radiation therapy. A strategy to tag hypoxic cells with luciferase protein Cells can be genetically tagged with marker proteins through site-specific recombination by Cre recombinase [32] , [33] , [34] . We generated a gene construct, CAGp/loxP-polyA-loxP-luciferase , that results in luciferase expression after Cre-mediated deletion of the poly A signal flanked by loxP sites ( Fig. 1a ). After co-transfection of the construct with CMVp-Cre that constitutively expresses Cre into human embryonic kidney 293 cells ( Fig. 1b , upper), luciferase was expressed regardless of oxygen tension ( Fig. 1c ). To generate a cell that would persistently express luciferase after experiencing hypoxia, we generated a hypoxia-inducible expression vector for Cre. We previously showed that HIF-1-dependent expression of arbitrary genes of interest could be obtained by a dual strategy, in which the artificial HIF-1-dependent promoter including 5 copies of HRE (5HREp) is responsible for the expression of a fusion protein composed of the product of a gene of interest and the ODD domain of HIF-1α [35] . The 5HREp/Cre–ODD gene, which expresses a Cre–ODD fusion protein under the control of HIF-1 ( Fig. 1b , middle), induced luciferase expression from CAGp/loxP-polyA-loxP-luciferase under hypoxic but not normoxic conditions ( Fig. 1c ). To add temporal specificity, we applied the Cre-ER T2 technique [32] , [33] , in which Cre-ER T2 translocates into the nucleus and induces site-specific recombination only in the presence of tamoxifen. We generated a construct, 5HREp/Cre-ER T2 –ODD ( Fig. 1b , lower), which expressed Cre-ER T2 –ODD under hypoxic conditions ( Fig. 1d ). The stable transfectant containing both CAGp/loxP-polyA-loxP-luciferase and 5HREp/Cre-ER T2 –ODD expressed detectable luciferase bioluminescence 16 h after tamoxifen treatment under hypoxic but not normoxic conditions ( Fig. 1e ). Estrogen did not induce luciferase activity under hypoxic conditions ( Fig. 1c ). Site-specific recombination was first detected at 16 h and peaked 24 h after tamoxifen treatment under hypoxia ( Fig. 1f ). Luciferase-tagging did not occur when HIF-1α expression was not fully induced either at 3% O 2 or under glucose-deprived conditions at 1 and 0.02% O 2 ( Supplementary Fig. S1a–c ). The luciferase-tagging was almost completely abrogated by HIF-1α downregulation ( Supplementary Fig. S1d–f ), or by treatment with a cell cycle inhibitor, hydroxyurea ( Supplementary Fig. S1g–i ). These results indicate that the luciferase-tagging was dependent on both HIF-1 activity and DNA replication. Taken together, these results document a tamoxifen-inducible luciferase-tagging strategy for HIF-1-active cells based on Cre-ER T2 /loxP site-specific recombination. 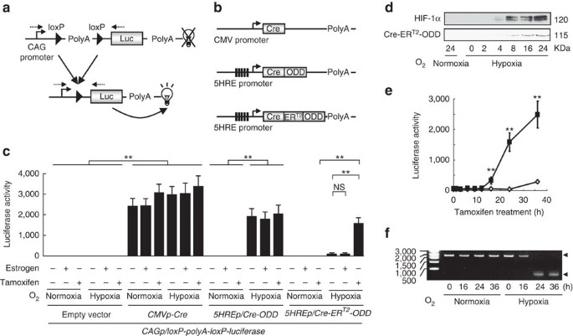Figure 1: Luciferase-tagging of hypoxic cells by HIF-1- and tamoxifen-dependent site-specific recombination. (a) Schematic diagram ofCAGp/loxP-polyA-loxP-luciferasegene (upper) that results in luciferase expression after Cre-mediated deletion of floxed poly A signal (lower). (b) Schematic diagrams ofCMVp-Cre(upper; expressing Cre constitutively),5HREp/Cre–ODD(middle; expressing Cre–ODD in a HIF-1-dependent manner),5HREp/Cre-ERT2–ODD(lower; expressing Cre-ERT2–ODD in a HIF-1-dependent manner) genes. (c) After transient transfection with the indicated gene constructs, cells were treated with (+) or without (−) estrogen or tamoxifen under normoxic or hypoxic conditions for 24 h and subjected to luciferase assay. Mean±s.d.n=3. The statistical significance of differences was determined using Student'st-test. **P<0.01. NS: not significant. (d) Stable transfectant with the5HREp/Cre-ERT2–ODDgene andCAGp/loxP-polyA-loxP-luciferasegene was treated with tamoxifen under normoxic or hypoxic conditions for the indicated period and subjected to immunoblotting using antibodies against HIF-1α, or the myc epitope tag for the Cre-ERT2–ODD fusion protein. (e) After normoxic (white rhombus) or hypoxic (black square) treatment for the indicated period, the stable cell was subjected to Luciferase assay. Mean±s.d.n=3. **P<0.01 (Student'st-test). (f) Genomic DNA was extracted after the same treatment as (e) and subjected to semi-quantitative genomic PCR assay. The sizes of the marker bands (base pair) are shown. The primers used in the PCR assay are shown in (a) as dotted arrows. Figure 1: Luciferase-tagging of hypoxic cells by HIF-1- and tamoxifen-dependent site-specific recombination. ( a ) Schematic diagram of CAGp/loxP-polyA-loxP-luciferase gene (upper) that results in luciferase expression after Cre-mediated deletion of floxed poly A signal (lower). ( b ) Schematic diagrams of CMVp-Cre (upper; expressing Cre constitutively), 5HREp/Cre–ODD (middle; expressing Cre–ODD in a HIF-1-dependent manner), 5HREp/Cre-ER T2 –ODD (lower; expressing Cre-ER T2 –ODD in a HIF-1-dependent manner) genes. ( c ) After transient transfection with the indicated gene constructs, cells were treated with (+) or without (−) estrogen or tamoxifen under normoxic or hypoxic conditions for 24 h and subjected to luciferase assay. Mean±s.d. n =3. The statistical significance of differences was determined using Student's t -test. ** P <0.01. NS: not significant. ( d ) Stable transfectant with the 5HREp/Cre-ER T2 –ODD gene and CAGp/loxP-polyA-loxP-luciferase gene was treated with tamoxifen under normoxic or hypoxic conditions for the indicated period and subjected to immunoblotting using antibodies against HIF-1α, or the myc epitope tag for the Cre-ER T2 –ODD fusion protein. ( e ) After normoxic (white rhombus) or hypoxic (black square) treatment for the indicated period, the stable cell was subjected to Luciferase assay. Mean±s.d. n =3. ** P <0.01 (Student's t -test). ( f ) Genomic DNA was extracted after the same treatment as ( e ) and subjected to semi-quantitative genomic PCR assay. The sizes of the marker bands (base pair) are shown. The primers used in the PCR assay are shown in ( a ) as dotted arrows. Full size image Luciferase-tagging of hypoxic cells in tumour xenografts To test the tagging strategy in vivo , we administered tamoxifen once to nude mice bearing subcutaneous tumour xenografts of the stable transfectant with 5HREp/Cre-ER T2 –ODD and CAGp/loxP-polyA-loxP-luciferase . Luciferase bioluminescence was detected on the first day after the single tamoxifen injection ( Fig. 2a,b ). Immunohistochemical staining of frozen tumour sections with both anti-HIF-1α antibody (red fluorescence) and anti-luciferase antibody (green fluorescence) detected the existence of cells with yellow colour, indicating co-localization of HIF-1α and luciferase proteins in regions distant from perfusion-positive blood vessels on the first day ( Fig. 2c–e ). Thus, this novel technology was able to tag HIF-1-active hypoxic cells with luciferase in a xenograft tumour after tamoxifen administration. We confirmed that treatment of cells with various acute/intermittent/cycling hypoxia in vitro , which induced transcriptional activity of HIF-1, as reported previously [36] , [37] , [38] , did not lead to luciferase-tagging because of the arrest of the cell cycle ( Supplementary Fig. S2 ), suggesting that the system efficiently tag perfusion-limited chronic hypoxia rather than acute hypoxia in vivo . Moreover, we revealed that the tamoxifen concentration in blood reached a maximum at 2 h after the drug's administration but dramatically decreased to about 10% by 24 h later ( Supplementary Fig. S3 ). The rapid clearance enabled us to specifically tag HIF-1-positive cells with luciferase in vivo at a precise window in time (approximately within 24 h after tamoxifen administration). 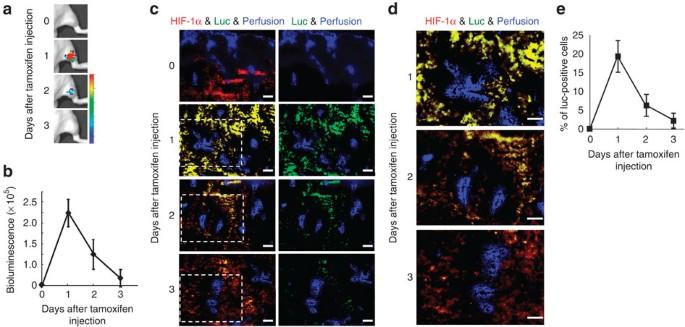Figure 2: Luciferase-tagging of hypoxic tumour cellsin vivo. (a) Optical imaging of mice bearing the tumour xenograft with the5HREp/Cre-ERT2–ODDgene andCAGp/loxP-polyA-loxP-luciferasegene at the indicated time points after the single administration of tamoxifen. Reproducibility was confirmed in ten independent mice, and representative images are shown. (b) Bioluminescent intensity in (a). Mean±s.d.n=10. (c) Immunohistochemistry with anti-HIF-1α (red) and anti-luciferase (green) antibodies of the tumour xenografts at the indicated times after the single injection of tamoxifen. Blue: Hoechst 33342 (perfusion marker). Bar, 50 μm. Yellow is merged green and red, indicating the co-localization of HIF-1α and luciferase proteins. (d) High magnification images of the enclosed areas inc. Bar, 50 μm. (e) Changes in the percentage of luciferase-positive cells in the tumour sections in (c) at the indicated time points after the single tamoxifen treatment, were calculated with NIH Image 1.63 (ref.29). Mean±s.d.n=20 fields in 5 independent sections. Figure 2: Luciferase-tagging of hypoxic tumour cells in vivo . ( a ) Optical imaging of mice bearing the tumour xenograft with the 5HREp/Cre-ER T2 –ODD gene and CAGp/loxP-polyA-loxP-luciferase gene at the indicated time points after the single administration of tamoxifen. Reproducibility was confirmed in ten independent mice, and representative images are shown. ( b ) Bioluminescent intensity in ( a ). Mean±s.d. n =10. ( c ) Immunohistochemistry with anti-HIF-1α (red) and anti-luciferase (green) antibodies of the tumour xenografts at the indicated times after the single injection of tamoxifen. Blue: Hoechst 33342 (perfusion marker). Bar, 50 μm. Yellow is merged green and red, indicating the co-localization of HIF-1α and luciferase proteins. ( d ) High magnification images of the enclosed areas in c . Bar, 50 μm. ( e ) Changes in the percentage of luciferase-positive cells in the tumour sections in ( c ) at the indicated time points after the single tamoxifen treatment, were calculated with NIH Image 1.63 (ref. 29 ). Mean±s.d. n =20 fields in 5 independent sections. Full size image Tracking the fate of hypoxic cells during tumour growth Because the site-specific recombination of our system occurs in the genomic DNA, the change will be inherited in all daughter cells, allowing us to follow the fate of tagged cells during tumour growth. After the tagging of HIF-1-active cells with luciferase on the first day after tamoxifen treatment, the number of luciferase-positive cells was reduced dramatically ( Fig. 2c–e ). To analyse the mechanism behind the reduction in more detail, we examined the spatio-temporal relationship between luciferase-tagged cells, HIF-1α-positive cells, and pimonidazole-positive cells over time ( Fig. 3a ). Double staining of sections with anti-HIF-1α and anti-pimonidazole antibodies showed that hypoxic regions were composed of two distinct areas: a HIF-1α-positive/pimonidazole-negative area (HIF-1-positive area) and a pimonidazole-positive/HIF-1α-negative area (pimonidazole-positive area). The HIF-1-positive area was closer to blood vessels, on average, than the pimonidazole-positive area in a tumour cord, consistent with previous reports [26] , [27] ( Fig. 3a,b ). It should be noted that HIF-1α is not usually expressed in perinecrotic/ischemic areas probably because of depletion of glucose at least in part ( Supplementary Fig. S1a ). Distances 'between pimonidazole-positive cells and blood vessels' and 'between HIF-1-positive cells and blood vessels' were constant over time, meanwhile that 'between luciferase-tagged cells and blood vessel' gradually increased during the observation ( Fig. 3a,b ). The luciferase-tagged cells were predominantly in the HIF-1-positive area and not in the pimonidazole-positive area on the first day after the single tamoxifen administration ( Fig. 3a,c ; Supplementary Fig. S4 ). On the second day, the tagged cells were mainly in the pimonidazole-positive area. On the third day, few tagged cells remained in the HIF-1- or the pimonidazole-positive areas, but some were found in necrotic regions. These results reveal a shift of tumour cells from the HIF-1-positive area to the pimonidazole-positive area, and further to necrotic regions during tumour growth. This represents a shift from moderately to severely hypoxic areas and explains why both luciferase bioluminescence ( Fig. 2a,b ) and luciferase-positive cells ( Fig. 2c–e ) dramatically decreased after the completion of luciferase-tagging in vivo . 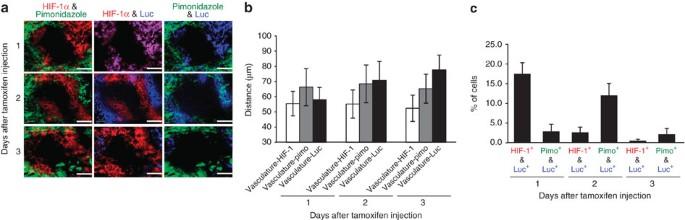Figure 3: Luciferase-tagging of hypoxic tumour cellsin vivo. (a) Immunohistochemistry with anti-HIF-1α (red), anti-pimonidazole (green), and anti-luciferase (blue) antibodies of tumour xenografts with the5HREp/Cre-ERT2–ODDgene andCAGp/loxP-polyA-loxP-luciferasegene at the indicated time points after the single injection of tamoxifen. *: Blood vessel. Bar, 50 μm. Reproducibility was confirmed in 12 independent sections. (b) Distances between vasculatures and HIF-1-positive cells (white), and pimonidazole-positive cells (grey), or and luciferase-tagged cells (black) were measured in the tumour sections in (a). Mean±s.d.n=40 tumour cords in 12 independent sections. (c) Percentages of cells detected with the indicated combination of antibodies in the tumour sections of (a) were quantified with CellSens Dimension (Olympus). Mean±s.d.n=40 tumour cords in 12 independent sections. Figure 3: Luciferase-tagging of hypoxic tumour cells in vivo . ( a ) Immunohistochemistry with anti-HIF-1α (red), anti-pimonidazole (green), and anti-luciferase (blue) antibodies of tumour xenografts with the 5HREp/Cre-ER T2 –ODD gene and CAGp/loxP-polyA-loxP-luciferase gene at the indicated time points after the single injection of tamoxifen. *: Blood vessel. Bar, 50 μm. Reproducibility was confirmed in 12 independent sections. ( b ) Distances between vasculatures and HIF-1-positive cells (white), and pimonidazole-positive cells (grey), or and luciferase-tagged cells (black) were measured in the tumour sections in ( a ). Mean±s.d. n =40 tumour cords in 12 independent sections. ( c ) Percentages of cells detected with the indicated combination of antibodies in the tumour sections of ( a ) were quantified with CellSens Dimension (Olympus). Mean±s.d. n =40 tumour cords in 12 independent sections. Full size image Survival of perinecrotic tumour cells after radiation therapy Applying the tagging technique, we examined the fate of each hypoxic fraction in tumour recurrence after radiation therapy. We irradiated tumours with a single dose of 25 Gy either 1 day after the single tamoxifen administration, when the tagged cells were mainly in the HIF-1-positive area or 2 days later when they were mainly in the pimonidazole-positive areas ( Fig. 3a,c ; Supplementary Fig. S4 ). At that dose, the tumours regressed and became non-palpable but later recurred ( Fig. 4a ). The bioluminescent intensity in the recurrent tumours was much higher when the radiation had been given to the xenograft in which tagged cells were located in the pimonidazole-positive area rather than HIF-1-positive area ( Fig. 4b,c ). Moreover, immunohistochemical analysis ( Fig. 4d,e ) and flow cytometric analysis ( Fig. 4f–h ) confirmed that there were more luciferase-tagged cells in the recurrent tumours after irradiation at 2 days, when the majority of the tagged cells were in the pimonidazole-positive area (57.4±9.9%) than at 1 day, when they were in the HIF-1-positive area (14.6±5.9%). Thus, the pimonidazole-positive tumour cells were more likely to survive radiation therapy. 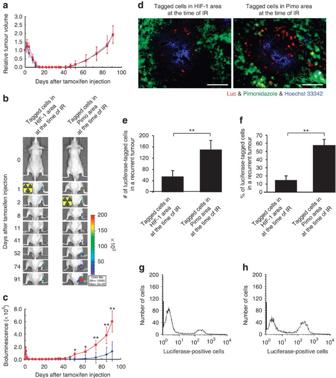Figure 4: Fate of hypoxic tumour cells after radiation treatment. (a) Tumour-bearing mice were γ-irradiated on either the first day after tamoxifen treatment when tagged cells were located in the HIF-1-positive cell area (blue rhombus; group name: tagged Cells in HIF-1 area), or the second day after tamoxifen treatment when the tagged cells were located in the pimonidazole-positive cell area (red square; group name: tagged cells in Pimo area). Relative tumour volume was calculated as the ratio of the tumour volume on each day to the corresponding volume on day 0. Mean±s.d.n=12. (b) During the experiment in (a), tumour-bearing mice were subjected to optical imaging at the indicated time points. Representative images are shown. (c) Bioluminescence intensities were quantified based on the optical imaging in (b). Blue rhombus: group of 'tagged cells in HIF-1 Area'. Red square: group of 'tagged Cells in Pimo area'. Mean±s.d.n=12. *P<0.05. **P<0.01 (Student'st-test). (d) The tumour xenografts in each group of the experiments (a–c) were surgically excised 91-days post-injection of tamoxifen and cut into two pieces. One of them was subjected to immunohistochemistry with anti-luciferase (red) and anti-pimonidazole (green) antibodies. Hoechst 33342: perfusion marker (blue). Bar, 50 μm. Reproducibility was confirmed in 40 tumour cords in 12 independent sections. (e) The number of luciferase-positive cells per tumour cord was counted in the tumour sections in (d). Mean±s.d.n=40 tumour cords in 12 independent sections. **P<0.01 (Student'st-test). (f) Single cell suspension was prepared from another piece of xenografts in (d) and subjected to flow cytometric analysis with anti-luciferase antibody to quantify percentage of luciferase-positive cells in the recurrent tumour of each group. Mean±s.d.n=12 independent tumour xenografts. **P<0.01 (Student'st-test). (g) Representative flow cytometric histogram in the 'tagged cells in HIF-1 area group'. Reproducibility was confirmed by using 12 independent xenografts. (h) Representative flow cytometric histogram in the 'tagged cells in Pimo area group'. Reproducibility was confirmed by using 12 independent xenografts. Figure 4: Fate of hypoxic tumour cells after radiation treatment. ( a ) Tumour-bearing mice were γ-irradiated on either the first day after tamoxifen treatment when tagged cells were located in the HIF-1-positive cell area (blue rhombus; group name: tagged Cells in HIF-1 area), or the second day after tamoxifen treatment when the tagged cells were located in the pimonidazole-positive cell area (red square; group name: tagged cells in Pimo area). Relative tumour volume was calculated as the ratio of the tumour volume on each day to the corresponding volume on day 0. Mean±s.d. n =12. ( b ) During the experiment in ( a ), tumour-bearing mice were subjected to optical imaging at the indicated time points. Representative images are shown. ( c ) Bioluminescence intensities were quantified based on the optical imaging in ( b ). Blue rhombus: group of 'tagged cells in HIF-1 Area'. Red square: group of 'tagged Cells in Pimo area'. Mean±s.d. n =12. * P <0.05. ** P <0.01 (Student's t -test). ( d ) The tumour xenografts in each group of the experiments ( a–c ) were surgically excised 91-days post-injection of tamoxifen and cut into two pieces. One of them was subjected to immunohistochemistry with anti-luciferase (red) and anti-pimonidazole (green) antibodies. Hoechst 33342: perfusion marker (blue). Bar, 50 μm. Reproducibility was confirmed in 40 tumour cords in 12 independent sections. ( e ) The number of luciferase-positive cells per tumour cord was counted in the tumour sections in ( d ). Mean±s.d. n =40 tumour cords in 12 independent sections. ** P <0.01 (Student's t -test). ( f ) Single cell suspension was prepared from another piece of xenografts in ( d ) and subjected to flow cytometric analysis with anti-luciferase antibody to quantify percentage of luciferase-positive cells in the recurrent tumour of each group. Mean±s.d. n =12 independent tumour xenografts. ** P <0.01 (Student's t -test). ( g ) Representative flow cytometric histogram in the 'tagged cells in HIF-1 area group'. Reproducibility was confirmed by using 12 independent xenografts. ( h ) Representative flow cytometric histogram in the 'tagged cells in Pimo area group'. Reproducibility was confirmed by using 12 independent xenografts. Full size image Because hypoxia is one of the most influential extrinsic factors to cellular radioresistance, we next examine the involvement of low oxygen concentration in radioresistance of pimonidazole-positive tumour cells. Immunocytochemistry in vitro showed that cells were stained with pimonidazole at less than 1% oxygen but not at 3% oxygen ( Supplementary Fig. S5 ); therefore, the pimonidazole-positive layer in a tumour cord would be under such oxygen conditions ( Table 1 ). Meanwhile, the HIF-1-positive layer seems to be exposed to relatively mild hypoxia at least 1–3% oxygen, because our site-specific recombination did not occur in the presence of 3% oxygen ( Supplementary Fig. S1a–c ), and because HIF-1-positive cells were not stained with pimonidazole in vivo ( Fig. 3a ). Taken together, pimonidazole-positive layers are under severer hypoxia than HIF-1-positive layers. Clonogenic cell survival assay showed that cells became more radioresistant under 0.02% severe hypoxia than 2% mild hypoxia ( Supplementary Fig. S6 ). Moreover, after radiation treatment, most cancer cells were stained with a DNA damage marker, γH2AX, in normoxic areas, but seldom in pimonidazole-positive areas ( Supplementary Fig. S7 ). All of these results indicate that the decreased oxygen concentration is responsible for the radioresistance of pimonidazole-positive cells at least in part. Table 1 Indirect characterization of the microenvironment in each layer of a tumour cord. Full size table HIF-1-dependent translocation of radio-surviving tumour cells We next analysed the tumour cells in the pimonidazole-positive area after irradiation in more detail. The xenografts were irradiated (25 Gy) 2 days after tamoxifen treatment when the tagged cells were in the pimonidazole-positive area and subjected to immunohistochemical analysis 4 days later ( Fig. 5a,b ). In the un-irradiated tumours, the luciferase-tagged cells almost completely disappeared ( Fig. 5b–d ), consistent with the shedding observed above ( Fig. 3 ). In contrast, in the irradiated tumours, tagged cells were present near perfusion-positive tumour blood vessels ( Fig. 5b,e,f : radiation (+) & HIF-1 inhibitor (−)). The same kind of results was confirmed in tumour xenografts of a human colon carcinoma cell line, WiDr ( Fig. 5g,h ). These results suggest that tumour cells in the pimonidazole-positive area translocated closer to the functional tumour blood vessels after surviving radiation. 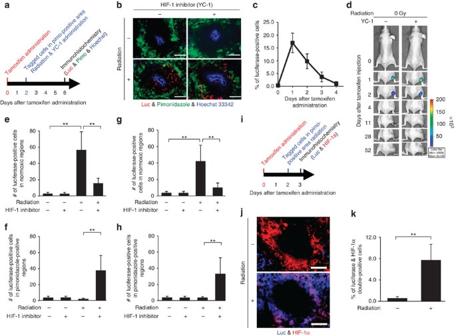Figure 5: Translocation of radio-surviving tumour cells. (a) Schematic diagram of treatments in (b). The tumour-bearing mice were treated with 0 (−) or 25 (+) Gy of γ-rays on 2 days after tamoxifen injection. YC-1 was administered to suppress radiation-induced activation of HIF-1 (ref.30). (b) Immunohistochemistry with anti-luciferase (red) and anti-pimonidazole (green) antibodies of the xenografts 4 days after the irradiation. Blue: Hoechst 33342. Bar, 50 μm. (c) The percentage of luciferase-positive cells on the indicated days was quantified in the unirradiated and DMSO-injected sections in (b).n=40 tumour cords in 12 sections. (d) The tumour-bearing mice were injected with (+) or without (−) YC-1 2 days after tamoxifen administration, and subjected to optical imaging on the indicated days. Representative images of 12 mice are shown. (e) The numbers of luciferase-positive cells in normoxic regions were quantified in the sections of (b).n=40 tumour cords in 12 sections. **P<0.01 (Student'st-test). (f) The numbers of luciferase-positive cells in pimonidazole-positive regions were quantified in the sections of (b).n=40 tumour cords in 12 sections. **P<0.01 (Student'st-test). (g) After transfection with the5HREp/Cre-ERT2–ODDgene andCAGp/loxP-polyA-loxP-luciferasegene, antibiotic-resistant WiDr cells were selected with blasticidin. Tumour xenografts, with the resultant stable transfectant, were subjected to the same experiment as (a,b). The numbers of luciferase-positive cells in normoxic regions were quantified in the sections.n=40 tumour cords in 12 sections. **P<0.01 (Student'st-test). (h) The numbers of luciferase-positive cells in pimonidazole-positive regions were quantified in the experiment of (g)n=40 tumour cords in 12 sections. **P<0.01 (Student'st-test). (i) Schematic diagram of treatments in (j). The tumour xenografts, with HEK293 transfectant, were subjected to immunohistochemistry 1 day following the 0 (−) or 25 Gy (+) of radiation. (j) Immunohistochemistry with anti-luciferase (blue) and anti-HIF-1α (red) antibodies. Bar, 50 μm. Representative images of 12 xenografts are shown. (k) Percentages of luciferase and HIF-1α double-positive cells were quantified in the sections of (j).n=40 tumour cords in 12 sections. **P<0.01 (Student'st-test). Figure 5: Translocation of radio-surviving tumour cells. ( a ) Schematic diagram of treatments in ( b ). The tumour-bearing mice were treated with 0 (−) or 25 (+) Gy of γ-rays on 2 days after tamoxifen injection. YC-1 was administered to suppress radiation-induced activation of HIF-1 (ref. 30 ). ( b ) Immunohistochemistry with anti-luciferase (red) and anti-pimonidazole (green) antibodies of the xenografts 4 days after the irradiation. Blue: Hoechst 33342. Bar, 50 μm. ( c ) The percentage of luciferase-positive cells on the indicated days was quantified in the unirradiated and DMSO-injected sections in ( b ). n =40 tumour cords in 12 sections. ( d ) The tumour-bearing mice were injected with (+) or without (−) YC-1 2 days after tamoxifen administration, and subjected to optical imaging on the indicated days. Representative images of 12 mice are shown. ( e ) The numbers of luciferase-positive cells in normoxic regions were quantified in the sections of ( b ). n =40 tumour cords in 12 sections. ** P <0.01 (Student's t -test). ( f ) The numbers of luciferase-positive cells in pimonidazole-positive regions were quantified in the sections of ( b ). n =40 tumour cords in 12 sections. ** P <0.01 (Student's t -test). ( g ) After transfection with the 5HREp/Cre-ER T2 –ODD gene and CAGp/loxP-polyA-loxP-luciferase gene, antibiotic-resistant WiDr cells were selected with blasticidin. Tumour xenografts, with the resultant stable transfectant, were subjected to the same experiment as ( a , b ). The numbers of luciferase-positive cells in normoxic regions were quantified in the sections. n =40 tumour cords in 12 sections. ** P <0.01 (Student's t -test). ( h ) The numbers of luciferase-positive cells in pimonidazole-positive regions were quantified in the experiment of ( g ) n =40 tumour cords in 12 sections. ** P <0.01 (Student's t -test). ( i ) Schematic diagram of treatments in ( j ). The tumour xenografts, with HEK293 transfectant, were subjected to immunohistochemistry 1 day following the 0 (−) or 25 Gy (+) of radiation. ( j ) Immunohistochemistry with anti-luciferase (blue) and anti-HIF-1α (red) antibodies. Bar, 50 μm. Representative images of 12 xenografts are shown. ( k ) Percentages of luciferase and HIF-1α double-positive cells were quantified in the sections of ( j ). n =40 tumour cords in 12 sections. ** P <0.01 (Student's t -test). Full size image It has been reported that radiation leads to reoxygenation of tumours and eventually upregulates HIF-1α expression. Molecular mechanisms behind this phenomenon are multiple: (1) enhanced translation of HIF-1α protein in a PI3K-Akt/mTOR-dependent manner [29] , [30] , and (2) stabilization of HIF-1α protein through the decrease in hydroxylation of Pro 402/564 by reactive oxygen [20] and through the S-nitrosylation of Cys 533 by NO generated in tumour-associated macrophages [39] . Taking advantage of the tagging technique, we examined whether the upregulation of HIF-1α expression was critical for the translocation of the pimonidazole-positive cells. First, we irradiated the xenograft when tagged cells were present in the pimonidazole-positive area, and performed immunohistochemistry the following day ( Fig. 5i,j ). The tagged cells disappeared in the non-irradiated tumour, but persisted and expressed HIF-1α in the irradiated tumour ( Fig. 5j,k ; Supplementary Fig. S8 ). In addition, we confirmed that inhibition of the radiation-induced upregulation of HIF-1 activity with the HIF-1 inhibitors, YC-1 ( Supplementary Fig. S9a,b ) [40] and Acriflavine [41] , dramatically reduced the translocation of the tagged cells ( Fig. 5b,e–h ; Supplementary Fig. S9c,d ) and suppressed tumour recurrence after radiation therapy ( Fig. 6a,b ). All of these results indicate that, after surviving radiation, perinecrotic tumour cells in the pimonidazole-positive area translocate to the proximal regions of tumour blood vessels in a HIF-1-dependent manner, leading to the initiation of tumour recurrence ( Supplementary Fig. S8 ). Finally, we examined possible involvement of epithelial–mesenchymal transition (EMT) in the translocation, because HIF-1 is known to provoke it and induce cell migration [42] , [43] . Increase in oxygen- and glucose-availability, which are known to activate HIF-1 in solid tumours after radiation therapy, shifted the expression of an epithelial marker (E-cadherin) to that of mesenchymal markers (vimentin and N-cadherin) in a HIF-1-dependent manner, suggesting the function of EMT in the translocation ( Supplementary Fig. S10 ). 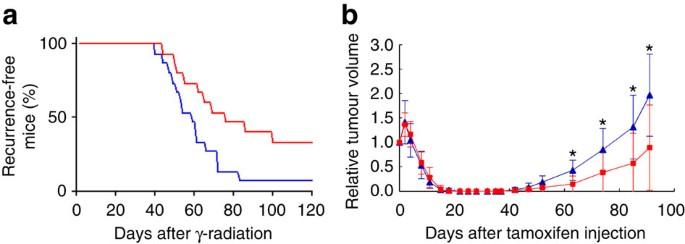Figure 6: Therapeutic effect of the combination of radiation and a HIF-1 inhibitor. (a) The tumour bearing mice were irradiated with γ-rays (25 Gy) and treated with or without YC-1 1 min after the irradiation to suppress the activation of HIF-1. Kaplan–Meier analysis of recurrence-free periods after irradiation alone (blue) or after the combination of radiation and a HIF-1 inhibitor (red).n=15. (b) During the experiment of (a), relative tumour volume was calculated as the ratio of the tumour volume on each day to the corresponding volume on day 0. Blue triangle: radiation alone group. Red square: radiation & YC-1 group. Mean±s.d.n=15. *P<0.05 (Student'st-test). Figure 6: Therapeutic effect of the combination of radiation and a HIF-1 inhibitor. ( a ) The tumour bearing mice were irradiated with γ-rays (25 Gy) and treated with or without YC-1 1 min after the irradiation to suppress the activation of HIF-1. Kaplan–Meier analysis of recurrence-free periods after irradiation alone (blue) or after the combination of radiation and a HIF-1 inhibitor (red). n =15. ( b ) During the experiment of ( a ), relative tumour volume was calculated as the ratio of the tumour volume on each day to the corresponding volume on day 0. Blue triangle: radiation alone group. Red square: radiation & YC-1 group. Mean±s.d. n =15. * P <0.05 (Student's t -test). Full size image In the present study, we established a novel system to tag hypoxic cells in a tumour xenograft at a specific window in time. Exploiting its advantages, we analysed the dynamics and fate of the cells during tumour growth and after radiation therapy. Here we successfully revealed that the pimonidazole-positive/HIF-1α-negative cancer cells (pimonidazole-positive cells) survive radiation better than their counterparts. Moreover, we demonstrate, for the first time, that the cells acquire high levels of HIF-1 activity in areas of radiation-induced reoxygenation and translocate towards tumour blood vessels after surviving radiation therapy. We previously reported that cancer cells which acquire HIF-1 activity after radiation treatment protect the tumour vasculature from the cytotoxic effects of radiation by inducing the expression of vascular endothelial cell-growth factor [30] . Here we identified pimonidazole-positive cells as the population that efficiently survive radiation and acquires significant HIF-1 activity. Taken together, these findings suggest that, by inducing HIF-1 activity, pimonidazole-positive cancer cells not only protect the tumour vasculature but also translocate towards the blood vessels, facilitating both indirectly and directly local tumour recurrence after radiation. The mechanisms behind the post-irradiation translocation of perinecrotic cells to regions close to blood vessels still remain unclear. Radiation-induced damage of normoxic cells generates a pressure gradient to the less damaged hypoxic region that might contribute to the translocation of the surviving cells. Alternatively, the hypoxic cells might actively migrate towards the blood vessels. Actually, we confirmed that the increase in oxygen- and glucose-availability, which are known to activate HIF-1 in solid tumours after radiation therapy, promoted EMT in a HIF-1-dependent manner ( Supplementary Fig. S10 ). The translocating cells would gain nutrients and oxygen through their proximity to the blood vessels, potentially facilitating tumour recurrence. The HIF-1-dependent translocation/migration of the surviving cells towards radio-protected blood vessels might suggest a novel function of HIF-1 in both local tumour recurrence and distant tumour metastasis after radiation therapy. To directly examine the involvement of HIF-1 in the post-irradiation translocation of perinecrotic cells, it was critical to inhibit the activation of HIF-1. Although the short interfering RNA technique is useful to specifically knockdown the expression of a target gene in general, we could not exploit it here because our tagging strategy is completely HIF-1-dependent ( Supplementary Fig. S1d–f ). Alternatively, we applied pharmacological inhibitors. Administration of the HIF-1 inhibitors, YC-1 ( Fig. 5b,e–h ) and acriflavine ( Supplementary Fig. S9c,d ), significantly suppressed the post-irradiation translocation of perinecrotic cells towards the vasculature. It is reasonable to conclude that these results were obtained through a common HIF-1-inhibiting effect, rather than a nonspecific/off-target effect, because the mechanisms of action of the drugs behind the HIF-1 blockade are completely different. To identify intratumoural localization of potential radio-surviving cells, it is critical to understand the characteristics of cells, which were tagged with luciferase through the HIF-1-dependent Cre-ER T2 /loxP system. It seems reasonable to assume that the tagged cells were under chronic hypoxia in the pimonidazole-positive sector, rather than acute hypoxia, because our in vitro data showed that treatment of cells with various acute/intermittent/cycling hypoxia, which induced HIF-1 activity [36] , [37] , [38] , did not promote luciferase-tagging ( Supplementary Fig. S2 ). If so, our finding that 57.4 (9.9%) of cells were tagged with luciferase in the recurrent tumour is somewhat surprising, because multiple studies have suggested the importance of acute rather than chronic hypoxia in tumour radioresistance [44] . However, we should not ignore the importance of acute hypoxia, because there remains a possibility that other acute hypoxic conditions, which we have not yet reproduced owing to its complexity [44] , [45] , could have induced luciferase-tagging in vivo . So, what were the origins of luciferase-negative cells detected in the recurrent tumours after radiation treatment had been given to the xenografts, in which tagged cells existed in the pimonidazole-positive sector? The origins seem to be multiple. One of the most reasonable answers is HIF-1-positive/luciferase-negative cells ( Supplementary Fig. S4 ). Another is acute/intermittent/cycling hypoxia because of the insufficient tagging of them. In addition, there is the possibility that normoxic tumour cells might have survived radiation and caused the luciferase-negative cells to some extent because the radioresistance under hypoxia is no more than three times that under normoxia [8] . Furthermore, we could not exclude the possibility that pimonidazole-positive/luciferase-negative hypoxia also caused the luciferase-negative cells in recurrent tumours because it is impossible to completely tag all of them with luciferase ( Supplementary Fig. S4 ). It is difficult to provide definitive answers because of the limitations of the tagging strategy. Exploiting the results of our study, we can characterize the microenvironments in each layer of a tumour cord ( Table 1 ). Pimonidazole-positive layer and HIF-1-positive layer seem to be under severe (<1% oxygen) and relatively mild (1–3% oxygen) hypoxia, respectively, as described above. The glucose-dependency of the luciferase-tagging in vitro ( Supplementary Fig. S1a-c ) suggests that HIF-1-positive cells, in contrast to pimonidazole-positive cells, are present under glucose-available conditions. The presence of hydroxyurea completely inhibited the luciferase-tagging in vitro ( Supplementary Fig. S1g-i ), suggesting that the HIF-1-positive cells are still proliferating. In the present study, we mainly used the HEK293 cell line that has no oncogenic mutations. This enabled us to assume that any phenomenon observed here was not dependent on oncogenic mutations and that most cells fundamentally have the ability to behave identically to the cells after radiation treatment. However, one needs to understand the potential disadvantages of using these cells. HEK293 is no more than an experimentally transformed cell line, and, therefore, would not be necessarily a good model for cancer research. From this point of view, we should not simply suppose that the phenomena/mechanism observed here would be general. Although we have confirmed a colon carcinoma cell line, WiDr, to have the same potential as HEK293 cells for tumour translocation ( Fig. 5g,h ), it is critical to further perform the same cell-tracking experiments using various cancer cell lines. Here we obtained enough information to understand how, when, and where 'the low pO 2 -mediated radiochemical mechanism' and 'the HIF-1-dependent radiobiological mechanism' function in response to radiation therapy. The predominant survival of pimonidazole-positive cells over the other populations can be simply explained by the radiochemical oxygen effect, because pO 2 critical for efficient DNA damage by ionizing radiation is extremely low [18] , [19] ( Table 1 ). Actually, the extent of DNA damage in pimonidazole-positive cells was not so severe compared with that in the other cells ( Supplementary Fig. S7 ). Following the survival, radiation-induced activation of HIF-1 is responsible for the translocation of the surviving cells towards tumour blood vessels, leading to tumour recurrence. On the basis of these findings, both radiochemical and radiobiological mechanisms should be inhibited for a better therapeutic effect. In addition to the HIF-1-dependent radiobiological mechanism, there are other biological processes that potentially affect radioresistance of hypoxic cells. It has been reported that hypoxia induces the expression of some cell cycle regulators [46] , [47] and eventually influences radiosensitivity of cells. Moreover, chronic hypoxia, but not acute hypoxia, decreases the expression of genes related to DNA damage repair and increases cellular radiosensitivity [48] , [49] . So, to fully elucidate molecular mechanism behind radioresistance of perinecrotic tumour cells, it is critical to further analyse spatiotemporal relationship among these biological processes in highly heterogeneous and dynamically changing tumour microenvironments during tumour growth and after radiation therapy. Cell culture and reagent The human embryonic kidney cell line (HEK 293) and human colon adenocarcinoma cell line (WiDr) were purchased from American Type Culture Collection. Cells were maintained in 10% FBS-Dulbecco's modified Eagle's medium. Normoxic and hypoxic conditions were achieved in a well-humidified incubator with 5% CO 2 and 95% air at 37 °C (O 2 =20%) and in a Bactron Anaerobic Chamber, BACLITE-2 (O 2 <0.02%; Sheldon Manufacturing), respectively. Hypoxic conditions with 1 and 3% were achieved in a hypoxic workstation, INVIVO 2 -500 (Ruskinn). Estrogen (17β-estradiol; Sigma-Aldrich) and tamoxifen (4-Hydroxytamoxifen; Sigma-Aldrich) were dissolved in ethanol, and YC-1 in DMSO. Doses of tamoxifen and YC-1 in vivo were 5 mg kg −1 and 100 mg kg −1 , respectively. Plasmid construct To construct the plasmid encoding 5HREp/Cre-ER T2 –ODD , the nuclear localization signal and luciferase gene in p5HRE–ODD-Luc [35] were substituted with a Cre recombinase (Cre)–estrogen receptor T2 (ER T2 ) fusion gene and myc epitope tag-coding sequence, respectively. To construct the plasmid encoding 5HREp/Cre–ODD , the nuclear localization signal and luciferase gene in p5HRE–ODD-Luc [35] were substituted with the Cre-coding sequence and myc epitope tag-coding sequence, respectively. To construct the plasmid encoding CMVp-Cre , which constitutively expresses Cre, the d2EGFP gene in pCMV-d2EGFP [50] was substituted with the Cre-coding sequence. To construct the plasmid encoding CAGp/loxP-polyA-loxP-luciferase , two loxP sites flanking the SV40 poly-adenylation signal were inserted downstream of the constitutively active chicken β-actin promoter (CAGp) of pCAG1. The coding sequence for the firefly luciferase gene was additionally inserted downstream. See Fig. 1a,b for schematic diagrams of the constructs. Stable transfectant HEK 293 cells were stably transfected with two plasmids encoding the 5HREp/Cre-ER T2 –ODD gene and the CAGp/loxP-polyA-loxP-luciferase gene, respectively, by the calcium phosphate method [51] . A representative clone, which showed HIF-1 and tamoxifen-dependent luciferase-tagging, was used in the present study. Luciferase-tagging experiments in vitro HEK 293 cells or their derivatives were seeded in 24-well plates (2×10 4 cells per well). For the experiment in Fig. 1c , the cells were transiently transfected with the indicated genes, and treated with estrogen or tamoxifen (100 nM) under normoxic (20% oxygen) or hypoxic (0.02% oxygen) conditions for 24 h. For the experiments in Fig. 1 d–f , the HEK293 stable transfectant was treated as described above. The cells were lysed with 100 μl of Passive lysis buffer (Promega) for luciferase assays using Luciferase assay reagent (Promega), according to the manufacturer's instructions. For genomic PCR assays, genomic DNA was purified with a MagExtractor genome kit (Toyobo), and 1 μg of DNA was subjected to PCR with a KOD Plus kit (Toyobo) and the primers, which annealed to the CAGp and luciferase-coding sequence as schematically represented in Fig. 1a . Sequences of primers are 5′-ctttgtcccaaatctggcggagccgaaatc-3′, and 5′-agcgtaagtgatgtccacctcgatatgtgc-3′. For immunoblotting, cell lysate was collected with 100 μl of 1×SDS–PAGE loading buffer, applied to SDS–PAGE, and reacted with anti-HIF-1α mouse monoclonal antibody (BD Bioscience; Working conc.=0.5 μg ml −1 ) and anti-myc-tag mouse monoclonal antibody (Cell Signaling Technology; ×2,000 dilution) for the detection of HIF-1α and Cre-ERT2–ODD, respectively. Proteins were detected using anti-mouse IgG horseradish peroxidase-linked whole antibody (GE Healthcare Bio-Science) and an ECL-PLUS system (GE Healthcare), according to the manufacturer's instructions. Luciferase-tagging of hypoxic tumour cells in vivo Stable cells (2×10 7 cells per 100 μL PBS) were subcutaneously transplanted into the right hind leg of immunodeficient mice (8-weeks old, male, BALB/c nu/nu; Shimizu Laboratory Supplies). For in vivo luciferase-tagging, the tamoxifen solution was injected once on day 0 into the footpad of the tumour-bearing right leg (5 mg kg −1 ). Radiation treatment in vivo The tumour xenografts were locally irradiated with 25 Gy of 137 Cs γ-rays using a Gammacell 40 Exactor (MDS Nordion International). Optical imaging of luciferase activity in tumour xenografts Optical imaging in vivo was carried out with an IVIS-200 (Caliper) [29] , [30] , [35] , [52] . Bioluminescent images were acquired just 3 min after the intravenous injection of the luciferin solution (200 μL of 5 mg ml −1 solution). During the imaging, the mice were anaesthetized with 2.5% isoflurane gas in the oxygen flow (1.5 L per min). Signal intensity was quantified and analysed using Living Image 2.50-Igor Pro 4.90 software (Caliper). Growth delay assay Tumour volume was calculated as 0.5×length×width 2 , and compared with the initial value to calculate relative tumour volume. Immunohistochemical analyses Tumour xenografts were surgically excised 90 min after an intraperitoneal injection with pimonidazole hydrochloride [6] (Natural Pharmacia; 60 mg kg −1 ) and 1 min after an intravenous injection with Hoechst 33342 (100 μl of 10 mg ml −1 solution; Invitrogen; especially in Figs 2c,d , 4d and 5b ). Frozen sections of the xenografts were prepared with OCT compound (Sakura Finetek). Immunostaining was performed with anti-HIF-1α antibody (BD Bioscience; Working conc.=2.5 μg ml −1 ), FITC-conjugated anti-pimonidazole mouse monoclonal antibody (Natural Pharmacia; ×100 dilution), and anti-luciferase goat polyclonal antibody (Promega; 500× dilution) in Tween-TBS buffer [29] , [30] . HIF-1α was detected with Alexa Fluor 546 rabbit anti-mouse IgG (Invitrogen; 2,000× dilution; Figs 2c,d , 3a and 5j ). Meanwhile, luciferase was detected with donkey anti-goat IgG conjugated with Alexa Fluor 350 (Invitrogen; ×2,000 dilution; in Figs 3a and 5j ), Alexa Fluor 488 (Invitrogen; 2,000× dilution; in Fig. 2c,d ), or Alexa Fluor 594 (Invitrogen; in Figs 4d and 5b ). The reproducibility of each staining was sufficiently confirmed by using enough number of sections (See each figure legend for details) and representative results are shown. FACS analyses To analyse the luciferase-positive fraction in recurrent tumours, 91 days after radiation treatment, tumour xenografts were surgically excised, minced and treated with a 0.25%. Trypsine solution for 20 min. The resultant single cell suspension was treated with DMEM containing 10% FBS, washed with PBS, and fixed in 4% paraformaldehyde-PBS. The cells were kept in a PST solution (PBS containing 4% Serum and 0.1% triton X-100) on ice for 15 min, then treated with anti-luciferase goat polyclonal antibody (Promega; 500× dilution) and Alexa Fluor 594 donkey anti-goat IgG (Invitrogen; 2,000× dilution) sequentially, and subjected to flow cytometry using FacsCalibur (BD Bioscience) equipped with a 15-mW argon laser in the FL1 (530/30) and FL2 (585/30) channels. Dead cells and debris were eliminated based on forward-angle and side-scatter. A total of 10,000 events were acquired per sample. Reproducibility was confirmed by using 12 independent tumour xenografts in each group and representative results are shown. Statistical analyses The statistical significance of differences was determined using Student's t -test. A P value <0.05 was considered to be significant. Ethics of animal experiments All animal experiments were approved by the Animal Research Committee of Kyoto University, and performed according to guidelines governing animal care in Japan. How to cite this article: Harada, H. et al . Cancer cells that survive radiation therapy acquire HIF-1 activity and translocate towards tumour blood vessels. Nat. Commun. 3:783 doi: 10.1038/ncomms1786 (2012).